Oxygen consumption rates in subseafloor basaltic crust derived from a reaction transport model Oceanic crust is the largest potential habitat for life on Earth and may contain a significant fraction of Earth’s total microbial biomass; yet, empirical analysis of reaction rates in basaltic crust is lacking. Here we report the first assessment of oxygen consumption in young (~8 Ma) and cool (<25 °C) basaltic crust, which we calculate from modelling dissolved oxygen and strontium pore water gradients in basal sediments collected during Integrated Ocean Drilling Program Expedition 336 to ‘North Pond’ on the western flank of the Mid-Atlantic Ridge. Dissolved oxygen is completely consumed within the upper to middle section of the sediment column, with an increase in concentration towards the sediment–basement interface, indicating an upward supply from oxic fluids circulating within the crust. A parametric reaction transport model of oxygen behaviour in upper basement suggests oxygen consumption rates of 1 nmol cm −3 ROCK d −1 or less in young and cool basaltic crust. Fluid flow through basaltic crust on mid-ocean ridge flanks has a significant role in cooling the Earth, regulating biogeochemical cycles within the oceans and providing chemical gradients (that is, between oxidizing seawater and reducing basaltic minerals) that offer potential for abiotic and biologically mediated electron transfer reactions [1] , [2] , [3] . The general pattern of fluid circulation within oceanic crust starts with deep seawater recharge at basaltic outcrops, thus supplying crustal aquifers with oxidants (for example, dissolved oxygen and nitrate) and other nutrients [4] , [5] , [6] . Such flow of entrained seawater through basaltic basement occurs within a range of crustal conditions, from acidic to basic, hot to cool and oxic to reducing [7] . The dynamics of many biogeochemical reactions within deep oceanic crust are not yet well understood, largely because of technical limitations in sampling an environment kilometres under water, buried beneath tens to hundreds of metres of sediment and comprising hundreds of metres of heterogeneous basaltic flows [7] , [8] . The ridge flank hydrothermal system on the eastern flank of the Juan de Fuca Ridge (JFR), where warm (65 °C), chemically reduced fluids circulate through basaltic basement [9] , [10] , is an oasis of data in what is otherwise a dearth of global data. Although the JFR system provides a highly reacted, warm end-member for studying basaltic basement biogeochemistry and microbial ecology [11] , [12] , [13] , the majority of the upper oceanic crust experiences much cooler (<20 °C) and presumably oxic conditions [2] . Relative to the warm JFR system, oxygen in cooler systems probably persists for longer periods of time, as abiotic removal of oxygen is sluggish kinetically [2] ; however, oxygen removal rates in oceanic crustal aquifers are unconstrained. As fluid circulates within basement formations, oxygen is consumed by abiotic or biotic reactions within the basaltic matrix, and some is lost to overlying sediment pore waters through diffusion where it is consumed by microbial respiration within the sediment [14] . Oxic conditions within subsurface basaltic crust have been implied by extrapolating oxygen profiles into upper basaltic basement from oligotrophic sediment recovered in the South and North Pacific Gyres [14] , [15] , [16] , and more recently from beneath the North Atlantic Gyre [17] , but the variation of basement concentrations and dynamics of oxygen consumption along a flow pathway within subsurface basaltic crust has not been described until now. North Pond is a sediment ‘pond’ (~13 × 7 km across) on the western flank of the Mid-Atlantic Ridge that overlies relatively young (~8 Ma) basaltic crust and has regional sediment accumulation up to 200 m in the valley between steep rocky outcrops of oceanic crust that rise up to 1.5 km above the pond. This site has been a focus of scientific ocean drilling for several decades [18] , [19] , [20] , [21] , [22] , [23] , [24] . Recent measurements of oxygen concentrations in the relatively shallow sediment draped near the edges of North Pond indicates a flux of oxygen from underlying basaltic crust, making the site a promising location for examining oxygen dynamics in upper basement. Here we show that oxygen is reactive in young and cool upper basaltic crust by using high-resolution oxygen concentration depth profiles through the complete sediment column to predict oxygen concentration in fluids that circulate within upper basaltic basement at North Pond. Modelling based on patterns of conservative tracer elements, principally strontium, resolves oxygen transport behaviour in upper basement. By using these two-dimensional fluid transport patterns and by separating the diffusive component from the reactive component, we derive estimates of oxygen consumption rates in upper basement in an effort to constrain potential vertically integrated metabolic rates in this subsurface oceanic crustal environment. Sediment oxygen and strontium profiles To examine the dynamics of oxygen within relatively young, cool upper basement, we measured dissolved oxygen concentrations in deep sediment drill cores collected through the entire sediment column to the basement at North Pond during Integrated Ocean Drilling Program (IODP) Expedition 336 (ref. 25 ). Our sampling locations overlap areas previously sampled by gravity coring, where oxygen profiles indicated a flux of oxygen from underlying basaltic crust into the relatively shallow sediment draped near the edges of North Pond [17] . We extended this analysis into thicker sediment sections using deep sea drilling methods that penetrated through the sediment–basement interface. Sediment sampled from four boreholes (Holes U1382B, U1383D, U1383E and U1384A; Fig. 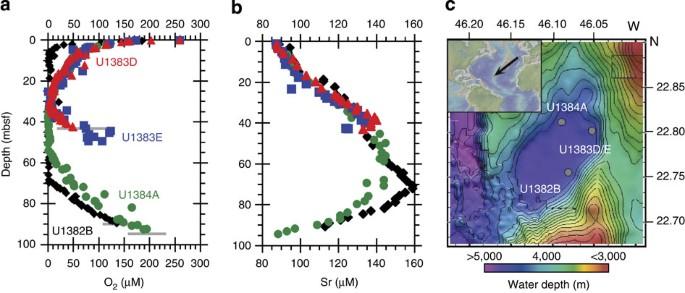Figure 1: Profiles of sediment oxygen and strontium concentrations at North Pond. Oxygen (a) and strontium (b) concentrations (in μM) in sediment collected from the western flank of the Mid-Atlantic Ridge during IODP Expedition 336 (map,c). Inaandb, depth (in m below seafloor (mbsf)) is indicated on the vertical axes, and black diamonds mark data from Hole U1382B; green circles, Hole U1384A; red triangles, Hole U1383D; and blue squares, Hole U1383E. Grey horizontal lines inaindicate basement depth at each hole, with the line crossing U1383D/E indicating basement depth at both holes. Inc, colour scale indicates water depth, ranging from 3,000 to 5,000 m depth, with contour lines at 100 m intervals. Location of coring sites are indicated with grey dots. Inset in upper left ofcindicates the location of the North Pond site in the North Atlantic Ocean. Map created using the default Global Multi-Resolution Topography Synthesis51basemap inGeoMapAppversion 3.2.1 (http://www.geomapapp.org). 1 , Table 1 ) ranges in thickness from 43.2 to 94.7 m below seafloor (mbsf) [25] . Sediments are predominantly nannofossil ooze with layers of coarse foraminiferal sand and occasional pebble-sized clasts of basalt, serpentinite, gabbroic rocks and bivalve debris [25] . Upper basement basalts are fresh-to-moderately altered, with typical mineralogical assemblages in alteration halos and veins such as clay minerals, Fe oxyhydroxide, carbonate and zeolite, reflecting predominantly oxic and seawater-dominated conditions [25] , as has been observed previously [26] . Figure 1: Profiles of sediment oxygen and strontium concentrations at North Pond. Oxygen ( a ) and strontium ( b ) concentrations (in μM) in sediment collected from the western flank of the Mid-Atlantic Ridge during IODP Expedition 336 (map, c ). In a and b , depth (in m below seafloor (mbsf)) is indicated on the vertical axes, and black diamonds mark data from Hole U1382B; green circles, Hole U1384A; red triangles, Hole U1383D; and blue squares, Hole U1383E. Grey horizontal lines in a indicate basement depth at each hole, with the line crossing U1383D/E indicating basement depth at both holes. In c , colour scale indicates water depth, ranging from 3,000 to 5,000 m depth, with contour lines at 100 m intervals. Location of coring sites are indicated with grey dots. Inset in upper left of c indicates the location of the North Pond site in the North Atlantic Ocean. Map created using the default Global Multi-Resolution Topography Synthesis [51] basemap in GeoMapApp version 3.2.1 ( http://www.geomapapp.org ). Full size image Table 1 Concentrations and fluxes of basement oxygen and strontium from IODP Expedition 336 Holes. Full size table Dissolved oxygen concentrations were measured using needle-type fibre-optic oxygen microsensors (see Methods). In all four of the North Pond boreholes, oxygen penetrates into the sediment column to a depth of 5–30 mbsf ( Fig. 1 ). All oxygen profiles have a characteristic ‘C’ shape, with high values near the seafloor, very low values within the middle portion of the sediment column and higher values close to the sediment–basement contact at depth. This pattern of O 2 concentrations indicates penetration of oxygen into the sediment from the seawater–sediment and the sediment–basement interfaces, defining distinct zones of oxic consumption within the sediment. These are the deepest sediment oxygen concentration measurements for the Atlantic Ocean, and only one site in the South Pacific Ocean (IODP Site U1371) has a documented non-zero dissolved oxygen concentration in deeper sediment [16] . Interstitial sediment pore water was collected and analysed using standard protocols (see Methods) to analyse the behaviour of other dissolved elements to establish which elements exhibit conservative (non-reactive) behaviour in this setting. Previously published profiles of other major ions (magnesium, calcium, potassium and sulphate) in the sediment are consistent with expectations for relatively shallow sediment and cool basement temperature (that is, relatively uniform with depth [18] , [27] ), whereas the profile of nitrate mirrors the oxygen profile [27] . Strontium was an element of interest because other investigations have demonstrated that fluid-rock Sr exchange is negligible at low temperatures in upper oceanic basement [28] , yet strontium is reactive in sediment, providing a discernable difference between sediment pore fluids and fluids that circulate within upper basement. Strontium concentrations in North Pond sediment pore waters display the typical increase with depth from carbonate diagenesis [29] until reaching a point where concentrations began to decrease towards seawater-like values at the upper basement because of diffusion of Sr out of the sediment and into basement ( Fig. 1 ), as has been observed previously at nearby Hole 1074A (ref. 18 ). The steepness of the gradients is a function of the degree of biogenic carbonate recrystallization within the sediment, in turn influenced by such factors as depositional rate, age and lithology of the sediment, and the Sr concentration in the basaltic basement aquifer. 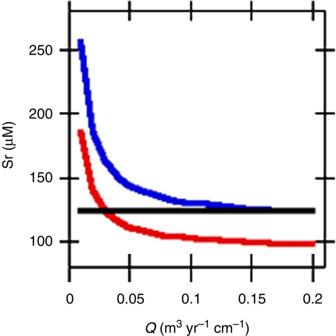Figure 2: Modelled versus predicted Sr concentrations in basement at various flow rates. A comparison of modelled Sr concentrations in upper basement at Hole U1383D (blue and red curves, respectively) versus the predicted concentrations from Hole U1383D (black line) for various assumptions of flow rate (QSW) between holes. The red and blue curves represent the Sr concentrations resulting from flow between Hole U1384A or Hole U1382B, respectively, and Hole U1383D. See Methods for more details on calculations. In addition, strontium isotopic composition of the North Pond sediment pore waters are virtually identical to modern seawater ( Table 2 ), confirming the non-reactivity of strontium in the basaltic portion of this system. If strontium reacted significantly within the basaltic basement in this setting, isotopic values would be much lower [30] . Thus, dissolved strontium is a measure of conservative exchange between basement fluid and sediment pore water in this setting, and offers a significant concentration gradient for accurate calculation of the diffusive transfer of ions between pore waters and basement fluids. Table 2 Isotopic composition of Sr in IODP Expedition 336 sediment pore waters. Full size table Reactive transport modelling of oxygen behaviour We use a reactive transport box model, described elsewhere [6] , [31] , to evaluate oxygen dynamics within basement at North Pond. This is done by calculating the diffusive flux across the sediment–basement interface from measured data; estimating the flow path, porosity and depth of the crustal reservoir; and then calculating fluid flux per unit width within basement. Diffusive fluxes across the sediment–basement interface and the concentrations of O 2 and Sr in upper basaltic basement are calculated from linear gradients in basal sediment concentrations at the depth of the sediment–basement interface (see Methods, Table 1 , Fig. 1 ). This assumes that the concentration of oxygen and strontium in upper basement is roughly equal to the basal sediment concentration, that the shallow basement aquifer is well mixed and that diffusion is the most important transport process between basement and sediment (that is, no advection into sediment from basement). Advection is unlikely to occur in the sediment, given the low permeability of the sediment column relative to the permeability of upper basaltic crust [32] . As sediment from Hole U1383E was highly disturbed with a relatively high degree of seawater contamination in pore fluids, especially at depth [27] , data from Hole U1383E are not included in further analyses. With the diffusive flux and the concentration of Sr in upper basaltic basement, volumetric fluid flux per unit width (that is, Q sw , calculated as described in the Methods) is then calculated between each of the sampled boreholes. Sr is used as the benchmark, as isotopic and concentration data indicate that Sr is non-reactive in the upper basement at this setting. This calculation results in estimated volumetric fluxes between each of the sampled boreholes of 0.03 and 0.19 m 3 yr −1 cm −1 , depending on the direction of flow from Hole U1384A or U1382B to U1383D, respectively ( Fig. 2 ). This range of rates is equivalent to or lower than similar fluxes calculated for the JFR flank [31] and the Dorado Seamount [6] , respectively. In the model, the values of Q sw range from 0.01 to 0.2 m 3 yr −1 cm −1 , spanning the range based on the Sr data. Figure 2: Modelled versus predicted Sr concentrations in basement at various flow rates. A comparison of modelled Sr concentrations in upper basement at Hole U1383D (blue and red curves, respectively) versus the predicted concentrations from Hole U1383D (black line) for various assumptions of flow rate ( Q SW ) between holes. The red and blue curves represent the Sr concentrations resulting from flow between Hole U1384A or Hole U1382B, respectively, and Hole U1383D. See Methods for more details on calculations. Full size image With these flux parameters, data for dissolved oxygen are inserted into the model to solve for the assumed concentration in upper basaltic basement, as described in the Methods. Differences between the model-calculated concentrations and those expected from linear extrapolation of the sediment pore water measurements must result from reaction, which are then solved for. The model-calculated oxygen values at Hole U1383D (that is, [O 2 ] end as described in the Methods) span the value predicted from extrapolating pore water profiles to the sediment–basement interface at Hole U1383D ( Fig. 3 ). For situations in which model calculations equal extrapolated concentrations (that is, where the line and curves cross), the decrease in dissolved oxygen is explained by losses due to diffusive exchange with sediment alone; however, this occurs at relatively low fluid fluxes (0.02 or 0.05 m 3 yr −1 cm −1 , depending on whether fluid flows from Hole U1384A or U1382B, respectively, to Hole U1383D; Fig. 3a,b ). These flow rates are lower than the flow rates predicted from the conservative tracer strontium (0.03 and 0.19 m 3 yr −1 cm −1 ; as indicated by vertical grey lines in Fig. 3 ). At the flow rates predicted from strontium data, the model oxygen concentrations are significantly higher at Hole U1383D than they are predicted to be from the basal sediment oxygen data. Oxygen consumption in upper basement must account for this difference. 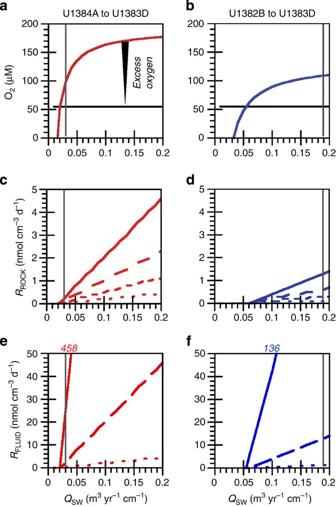Figure 3: Results of transport model of oxygen dynamics in basement. Panelsaandbcompare the modelled upper basement oxygen concentrations (μM) of Hole U1383D (red curve inaand blue curve inb) with the predicted upper basement concentration at this Hole (black lines). Curves are calculated with input concentrations predicted for upper basement from Holes U1384A and U1382B, respectively, across a range of possible flow rates,QSW(in m3yr−1cm−1), assuming oxygen is removed from transport processes only (see text for further details about the model). The vertical grey lines represent the predicted volumetric flow rates (Q) for fluids moving from Holes U1384A and U1382B, respectively, calculated from basal sediment strontium fluxes (see text). The difference between the red or blue curves and the predicted oxygen concentrations (black lines) for Hole U1383D in panelaandbindicate an excess of oxygen that would require another removal process, such as oxygen consumption. Panelscanddshow the range of calculated bulk rates of oxygen removal in rock (nmol O2cm−3ROCKd−1) needed to balance the modelled and predicted oxygen concentrations in upper basement assuming flow to Hole U1383D from Holes U1384A or U1382B, respectively. In these panels, lines represent scenarios where the reactive zone occurs only in the upper 50 m (solid line), 100 m (longer-dashed line), 200 m (medium-dashed line) or 500 m (small-dashed line) of basement. The lower panelseandfpresent the fluid oxygen consumption rates (nmol O2cm−3FLUIDd−1) calculated with porosity of basement taken into account, ranging from end-member scenarios of 50-m-thick reaction zones with 1% porosity (solid lines), 50 m with 10% porosity (long-dashed line, equivalent to 500 m with 1% porosity) and 500 m with 10% porosity (small-dashed line). Note that the ‘50m 1%’ porosity scenario generates rates of consumption higher than the axis range, with the reaction rate indicated by the italicized values outside panelseandf(that is, 458 and 136) for aQ-value of 0.2 m3yr−1cm−1. Figure 3: Results of transport model of oxygen dynamics in basement. Panels a and b compare the modelled upper basement oxygen concentrations (μM) of Hole U1383D (red curve in a and blue curve in b ) with the predicted upper basement concentration at this Hole (black lines). Curves are calculated with input concentrations predicted for upper basement from Holes U1384A and U1382B, respectively, across a range of possible flow rates, Q SW (in m 3 yr −1 cm −1 ), assuming oxygen is removed from transport processes only (see text for further details about the model). The vertical grey lines represent the predicted volumetric flow rates ( Q ) for fluids moving from Holes U1384A and U1382B, respectively, calculated from basal sediment strontium fluxes (see text). The difference between the red or blue curves and the predicted oxygen concentrations (black lines) for Hole U1383D in panel a and b indicate an excess of oxygen that would require another removal process, such as oxygen consumption. Panels c and d show the range of calculated bulk rates of oxygen removal in rock (nmol O 2 cm −3 ROCK d −1 ) needed to balance the modelled and predicted oxygen concentrations in upper basement assuming flow to Hole U1383D from Holes U1384A or U1382B, respectively. In these panels, lines represent scenarios where the reactive zone occurs only in the upper 50 m (solid line), 100 m (longer-dashed line), 200 m (medium-dashed line) or 500 m (small-dashed line) of basement. The lower panels e and f present the fluid oxygen consumption rates (nmol O 2 cm −3 FLUID d −1 ) calculated with porosity of basement taken into account, ranging from end-member scenarios of 50-m-thick reaction zones with 1% porosity (solid lines), 50 m with 10% porosity (long-dashed line, equivalent to 500 m with 1% porosity) and 500 m with 10% porosity (small-dashed line). Note that the ‘50m 1%’ porosity scenario generates rates of consumption higher than the axis range, with the reaction rate indicated by the italicized values outside panels e and f (that is, 458 and 136) for a Q -value of 0.2 m 3 yr −1 cm −1 . Full size image A reaction term is invoked in the model to account for removal of oxygen in upper basement along a flow path not accounted for by the diffusive model (see Methods for model equations). This parametric model has several simplifying assumptions. First, it is assumed that fluids within uppermost basement (<500 m below the sediment–basement interface) are connected, porous (1–10% pore space) and well mixed [6] , [23] . Second, it is assumed, yet well justified, that oxygen transport across the sediment–basement interface is strictly controlled by diffusion because the permeability in basement is orders of magnitude greater than that in overlying sediment and driving forces are minimal [33] . These assumptions have been used elsewhere to determine the sediment–basement interface fluxes on ridge flanks and near basement outcrops [6] , [31] . Third, the model assumes a flow direction between holes based on the relative changes in Sr concentrations in basement fluids (that is, from Hole U1384A or U1382B to Hole U1383D). As the underlying hydrogeology of North Pond is speculative [17] , the model assumptions of direct flow between sites represents a modest uncertainty on the scale of uncertainties associated with crustal conditions. Moreover, by focusing on the chemical, rather than the geophysical patterns of the basement aquifer, the direction of flow becomes less important than the residence time of the fluids and the resulting geochemical patterns that are produced. Although basement topography undoubtedly varies between holes, and there is a nominal height difference of roughly 50 m between holes ( Table 1 ), the box model considers an average condition along a length of transport that is orders of magnitude larger than vertical height differences. The calculated volumetric fluxes can be considered minimums, as they represent direct flow from one borehole to another, whereas the actual pathway of the fluids is likely tortuous in both horizontal and vertical directions. Figure 3c,d presents the range of bulk rock oxygen consumption rates for various thicknesses of upper basement, ranging from 50 to 500 m. The modelled rates ranged from 0.01 to almost 5 nmol O 2 consumed cm −3 ROCK d −1 cm −1 . Assuming the fluid flow rates estimated from the Sr data (indicated by vertical grey lines in Fig. 3 ), the bulk rock reaction rates are <1 nmol cm −3 d −1 cm −1 ( Fig. 3c,d ). If average porosity of basement is taken into account (assumed to range from 1 to 10%), confining the reactive space to the fluids within the rock matrix, then the associated modelled oxygen consumption rates range from 0.1 to ~100 nmol O 2 consumed cm −3 FLUID d −1 ( Fig. 3e,f ). If flow rates were similar to those estimated for the JFR flank system [34] (that is, ~0.2 m 3 yr −1 ), then oxygen reaction rates of nearly 500 nmol O 2 consumed cm −3 FLUID d −1 can be supported. Considering that oceanic crust may be the largest reservoir for microbial life on Earth, it is imperative to estimate rates of biogeochemical reactions in this system to understand the energy available that could support microbial activity. It is exceedingly difficult, however, to directly measure oxygen concentrations (let alone reaction rates) in upper basement because of technical limitations in accessing this environment. As a proxy, we use basal sediment oxygen concentrations ( Fig. 1 , Table 1 ) to predict the behaviour of oxygen in upper basement by way of a conservative reaction transport model. Model calculations indicate that oxygen concentrations along an assumed flow path should be higher than they are estimated from basal sediment pore water profiles ( Fig. 3a,b ), requiring a reactive term for balance. Constraining fluid flow rates with values predicted from the non-reactive behaviour of strontium in this system ( Fig. 2 ) results in rates of oxygen removal that are ~1 nmol cm −3 ROCK d −1 or less ( Fig. 3c,d ), depending on the presumed depth and porosity of upper basement in the model system. These are the first predictions of oxygen removal rates within basaltic basement. Although indirect, the model is appropriate, as it is based on established principles regarding the usage of basal sediment pore water concentration data to determine upper basement fluid concentrations built from long-term and repeated observations on the JFR crustal system, where pore water extrapolations are directly compared with natural borehole formation fluid compositions [5] , [34] , [35] , [36] . Similar models have also been applied to explain transport-reaction behaviour in other seafloor systems [6] . Our reliance on strontium as a conservative element in this system with respect to fluid reaction in upper basaltic crust is similar to the use of lithium concentration and isotopic data in another model system [36] . The largest unknown variable within this model is volumetric fluid flux within basement. In the North Pond system, heat flow data and seafloor observations suggest [17] that seawater recharges the system around the southern or western rim of North Pond, circulates underneath the sediment pond and then discharges along the northern and eastern edges. This general flow path of south-north/west-east flow is consistent with higher heat flow values to the north [37] , regional geological trends showing major fault systems, and typical structures generated by the spreading center to the east, which lies in a south/north orientation. However, the magnitude of flow in this region is poorly constrained. We present our model across a range of flow rates that have been estimated for other systems, and that correspond to rates predicted from the modelled behaviour of the conservative tracer strontium, to derive conservative rate estimates of oxygen consumption in upper basement. In other basement systems, values up to 1,800 m 3 yr −1 cm −1 have been estimated from the flux of conservative tracers across the sediment–basement interface, although that result is thought to be the highest volumetric flux currently observed in any subseafloor aquifer [6] , [31] . The calculated oxygen consumption rates in upper basement have important implications for global oxygen consumption in the ocean crust. It is estimated from rock alteration studies that ~10 12 mol iron and ~10 11 mol sulphur are oxidized by oxygen (and some nitrate) per year in relatively young (<20 Ma) upper (500±200 mbsf) oceanic crust [2] . Globally, this translates to an average iron oxidation rate of ~700 μmol Fe cm −3 (rock) yr −1 . These oxidation rates are several orders of magnitude higher than the oxygen consumption rates predicted here by using conservative basement fluid flow rates ( Fig. 3c,d ). Even taking into account the 4:1 stoichiometry of iron oxidized to oxygen reduced, the corresponding oxygen consumption rate needed to balance the estimates of crustal iron oxidation is many orders of magnitude higher than our calculations suggest. As mentioned previously, our estimates of oxygen consumption are likely minimums, as the fluid flow pathway is likely significantly more tortuous than our model assumes, which would result in a longer residence of seawater-derived fluids in basement. Moreover, considering the heterogeneous hydrology of basement, our estimates of oxygen consumption based on measurements from the sediment–basement interface may not be representative of rates of reaction through the entire upper section of hydrologically active basement of roughly 500 m depth. Thus, it is likely that higher oxygen consumption rates will be indicated once fluid flow rates and paths are better constrained. Our analysis does not allow us to discern between abiotic and biotic consumption within the crust; however, given the kinetic favourability of biotic oxidation of iron and sulphide in this cool ridge flank system [2] , it is likely that a significant fraction of the predicted oxygen consumption is biotic in nature. Recent studies have documented the presence of active microbial communities in the JFR flank setting [11] , [13] , [38] , although this is a warm and chemically reduced environment that is not representative of global upper crustal conditions. Confirmation of oxygen consumption by active microbial communities in cool temperature (<25 °C) upper oceanic crust still remains to be done. The reaction transport model used here is an oversimplification of fluid flow in this system, considering the three-dimensional nature of basement topography; however, the model is useful for constraining oxic consumption rates in young upper basement. Evaluation of the magnitude and direction of fluid flow within the basement at North Pond is currently underway, taking advantage of long-term-coupled hydrogeological, chemical and microbial observatories installed in deep crust at North Pond [25] . Further, direct measurements of oxygen concentrations in the formation fluids at North Pond will make it possible to validate these model predictions, assuming fluids in the borehole observatories return to pre-drilling conditions over the next several years. Analysis of crustal materials recovered during IODP Expedition 336 and those deployed within the observatories themselves should provide complimentary information on the presence, abundance, diversity and function of microbial communities harboured in deep basaltic crust. Sediment collection Procedures for sediment and basement coring during the expedition are described in more detail elsewhere [25] . Four holes (that is, Holes U1382B, U1383D, U1383E and U1384A) were cored at three different site locations within North Pond during the expedition; however, sediment from Hole U1383E was highly disturbed, with a relatively high degree of seawater contamination in pore fluids [27] . Thus, data from Hole U1383E were not included in modelling analyses. At each hole, the entire sediment column was Advanced Piston Corer cored until basement contact, with subsequent extended core barrel coring of the upper basement interval. Hole U1382B, the southernmost sediment hole, is located midway (about 25 m) between Holes 395A and U1382A, both of which are basement-penetrating holes with instrumented observatories [27] . Hole U1383D is located in the northeastern quadrant of the pond, about 5.9 km from Site U1382; this hole is about 10−15 m away from Holes U1383B and U1383C, which are also basement-penetrating instrumented holes [27] , [39] . Hole U1384A was cored in the northwestern side of the pond, being roughly 3.9 and 6.2 km away from the other sites (Holes U1383 and U1382, respectively). As described elsewhere [25] and consistent with thinner sediment cores from the region [17] , [40] , the sediments at all locations consisted of light brown to brown nannofossil ooze with layers of foraminiferal sand, with the lower few metres of each sediment column near the sediment–basement interface transitioning from a dark brown to rusty-coloured clay sediment. The sandy layers show erosional bases and fining-upwards sequences, indicating turbidite deposits. Visual observation as well as detection of fluorescent microsphere contamination tracers within sediment samples revealed that many of the sandy layers were highly disturbed during the core recovery. Oxygen measurements Following removal of whole-round core and syringe samples on the catwalk for microbiological sampling and pore water collection (up to 36% of core recovered was removed [25] ), all remaining core sections were capped and immediately transferred to the ship’s hold deck-refrigerated storage area for oxygen profiling, similar to the procedure followed during IODP Expedition 329 (refs 16 , 41 ). The cold storage area was maintained at roughly 6 °C throughout the sampling period, and cores were typically delivered to cold storage within 45 min of receiving them on the deck. Oxygen was measured by using needle-type fibre-optic oxygen microsensors (optodes; PreSens, Regensburg, Germany [42] ), inserted manually into sediments through holes drilled in the core liners. Temperature was measured within 2 cm of the oxygen-sampling location. Both optode and temperature sensors were connected to a MICROX TX3 single channel fibre-optic oxygen meter, which was calibrated according to the manufacturer’s protocols (PreSens). The reliable limit of detection was roughly 5 μmol l −1 . Some sections could not be profiled because of high sediment disturbance or inclusion of rocks within the sediment matrix. Strontium concentration and isotopic measurements Interstitial water samples were obtained from 10 to 20 cm length whole-round cores cut on the catwalk using standard procedures, as outlined elsewhere [43] . Splits of the fluid samples were acidified with 4 ml of sub-boiled 6 mol l −1 HCl per litre sample for shore-based analysis of Sr concentrations using inductively coupled plasma-optical emission spectroscopy. Splits of the fluid samples, corresponding to about 1 μg of Sr, were evaporated to dryness on a hot plate and dissolved in 0.5 ml of sub-boiled 3 mol l −1 HNO 3 . Sr was subsequently separated by using a 0.2-ml column of Sr-Spec, a Sr-selective extraction chromatographic resin [44] , [45] produced by Eichrom Technologies, Inc. The sample was loaded onto the column and the matrix was subsequently washed with 2.5 ml of 3 mol l −1 HNO 3 . Sr was then eluted using 4 ml of 0.01 mol l −1 HNO 3 , dried down and dissolved in 2 ml of 0.28 mol l −1 HNO 3 . Sr isotope ratio analyses were undertaken using the Thermo Fisher Scientific Neptune MC-ICP-MS operated at IFREMER. An aliquot of a Sr isotope standard SRM 987 was measured every two samples to evaluate the reproducibility and accuracy of the instrument. The data were corrected for mass fractionation using an exponential law and 86 Sr/ 88 Sr=0.11935. Twenty-five analyses of the NIST SRM 987 standard made during the course of analyses have a mean value of 87 Sr/ 86 Sr=0.71034±3 (2s). Seawater reference materials CASS4 and NASS5 (NRC Institute for National Measurement Standards) were also analysed along with the samples; we obtained 87 Sr/ 86 Sr=0.70918±4 (2s, n =3) and 87 Sr/ 86 Sr=0.70919±9 (2s, n =3), respectively. Calculating basement conditions and rates The sediment oxygen and strontium profiles were used to calculate diffusive fluxes into the sediment from overlying water and from basement using Fick’s first law of diffusion [46] . The diffusive flux was calculated in two different ways. In the first method, the gradients below the sediment surface and above the sediment–basement interface were calculated by linear fitting of the data (excluding any obvious outliers in the data, interpreted to result from sediment disturbance). The surface oxygen gradients were calculated from the four uppermost data points, which ranged from 10 to 407 cm below sea floor. The oxygen diffusive flux was then calculated from the gradients using the following equation: where φ equals the sediment porosity, D sed is the diffusion coefficient for oxygen in sediments and δ[O 2 ]/δ z equals the change in oxygen concentration with depth (that is, the gradient calculated above), as described elsewhere [47] . The sediment porosity was calculated from bulk moisture and density measurements made on board the ship, using standard protocols [25] . The average sediment porosity for all sediments was 64.1±2.9 volume%, which corresponds well to porosity values obtained from shallower sediments in the region [17] . The diffusion coefficient for oxygen in sediment was calculated from the molecular diffusion coefficient of oxygen in free solution (1.13 × 10 −9 m 2 s −1 (ref. 48 )), corrected for in situ salinity and temperature [48] . The in situ temperature was assumed to be 1.5 °C for the surficial sediments and 5 °C for the basal sediments, based on upper basement temperature profiles from the region [23] , [24] . A similar equation was developed for calculating the strontium flux, where the diffusion coefficient for strontium [48] was 451.1 cm 2 yr −1 . In the second method, the flux of oxygen was calculated using PROFILE [49] . The sediment oxygen data were divided into two units to improve modelling fits—a surface unit consisting of the surficial data down to a depth where oxygen concentrations reached zero, and a basal unit consisting of the data from where oxygen concentrations were zero down to the deepest sample. To model the surface data, the boundary conditions were set to a bottom oxygen concentration of zero and a bottom oxygen flux of zero. The water column oxygen concentration was assumed to be 250 μmol l −1 , which agrees well with a value of 259 μmol l −1 recently reported for bottom water at this site [17] . To model the basal sediment oxygen data, the boundary conditions were set to a top flux of zero and the assumed basement oxygen concentration. The diffusion coefficient for oxygen in solution was calculated as above [47] , and the sediment diffusion coefficient was calculated by assuming that sediment diffusion is the product of the diffusion coefficient in solution divided by (1 × 3(1− φ )). Similar to the box model used elsewhere [6] , the model was defined by the length between two sediment holes (that is, between U1382B and U1383D, 5.9 km or between U1384A and U1383D, 3.9 km), with a cross-section of 1 × 1 cm 2 . The input concentration into the box is the basement oxygen concentration at one hole ([O 2 ] start ), calculated as described above. The concentration of oxygen at basement at the terminus of the box model ([O 2 ] end ) is determined assuming only diffusive removal of oxygen across the sediment–basement interface and advective transport of oxygen along the flow path, according to the following equation: where F a equals the advective flux of oxygen (in units of μmol yr −1 cm −1 width), F d equals the diffusive flux of oxygen from basement into sediment perpendicular to the flow path and Q sw equals the volumetric flux of fluid within basement (m 3 yr −1 cm −1 ). The diffusive flux parameter is taken from the values calculated from the basal sediment oxygen profiles, as described above. The advective flux is calculated as A similar model was developed using the strontium data to constrain the advective flow rate term ( Q sw ). As Sr behaves conservatively in this environment, the reactive flux can be set to zero, and Q sw can be solved based on the diffusive flux alone. Any difference between the modelled and assumed basement oxygen concentration is because of reactive processes within basement, where the rate of reaction ( R , in μmol yr −1 cm −1 ) is calculated as In this equation, X represents the distance between the start and end points (that is, between U1382B and U1384A). A volumetric rate of reaction is calculated by dividing R by the assumed depth of reaction in upper basement (assumed to range from 50 to 500 m) and further correcting for the porosity of the rock (1–10%). How to cite this article: Orcutt, B. N. et al. Oxygen consumption rates in subseafloor basaltic crust derived from a reaction transport model. Nat. Commun. 4:2539 doi: 10.1038/ncomms3539 (2013).